Charge order and its connection with Fermi-liquid charge transport in a pristine high-Tccuprate Electronic inhomogeneity appears to be an inherent characteristic of the enigmatic cuprate superconductors. Here we report the observation of charge–density–wave correlations in the model cuprate superconductor HgBa 2 CuO 4+ δ ( T c =72 K) via bulk Cu L 3 -edge-resonant X-ray scattering. At the measured hole-doping level, both the short-range charge modulations and Fermi-liquid transport appear below the same temperature of about 200 K. Our result points to a unifying picture in which these two phenomena are preceded at the higher pseudogap temperature by q =0 magnetic order and the build-up of significant dynamic antiferromagnetic correlations. The magnitude of the charge modulation wave vector is consistent with the size of the electron pocket implied by quantum oscillation and Hall effect measurements for HgBa 2 CuO 4+ δ and with corresponding results for YBa 2 Cu 3 O 6+ δ , which indicates that charge–density–wave correlations are universally responsible for the low-temperature quantum oscillation phenomenon. Charge–density–wave (CDW) correlations within the quintessential CuO 2 planes have been argued to either cause [1] or compete with [2] the superconductivity in the cuprates, and they might furthermore drive the Fermi-surface reconstruction in high magnetic fields implied by quantum oscillation (QO) experiments for YBa 2 Cu 3 O 6+ δ (YBCO) (ref. 3 ) and HgBa 2 CuO 4+ δ (Hg1201) (ref. 4 ). Consequently, the observation of bulk CDW order in YBCO was a significant development [5] , [6] , [7] . Hg1201 features a particularly simple crystal structure and has been demonstrated to exhibit Fermi-liquid charge transport in the relevant temperature-doping range of the phase diagram, whereas for YBCO and other cuprates, this underlying property of the CuO 2 planes is partially or fully masked [8] , [9] , [10] . It therefore is imperative to establish whether the pristine transport behaviour of Hg1201 is compatible with CDW order. 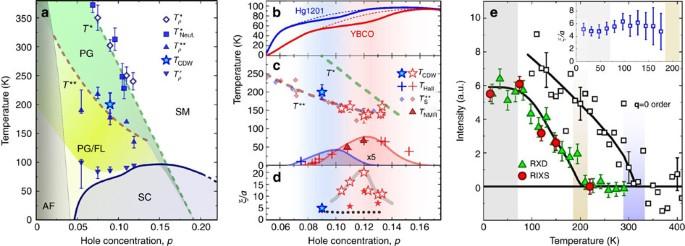Figure 1: Phase diagram. (a) Phase diagram of Hg1201. Blue line:Tc(p) (ref.13). Blue symbols: pseudogap (PG) temperatureT*, determined from the deviation from linear-Tresistivity in the ‘strange’ metallic (SM) regime and from the onset ofq=0 magnetism11,12. Yellow area: Fermi-liquid (FL) regime betweenT** and the measureable onset of superconducting (SC) fluctuations atTρ′. Grey area: estimated extent of antiferromagnetic (AF) phase. Since data belowp=0.05 are unavailable for Hg1201, the phase diagram is extended top=0 as in ref.8based on results for YBCO.Supplementary Fig. 1bshows comparison with YBCO. Characteristic transport temperatures are from ref.8and from additional measurements (see Methods). The error bar ofTCDWis estimated from the CDW peak onset and marked as a brown band ine. (b) Solid lines:Tc(p) for Hg1201 (ref.13) and YBCO14. Dashed lines: hypothetical ideal (approximately parabolic) ‘superconducting domes.’ (c) Solid lines: deviation of the SC dome from ideal shape (multiplied by 5);p=0.09 for Hg1201 corresponds top=0.11–0.12 for YBCO. Crosses: temperatures at which the Hall coefficient changes sign in high magnetic field20. Red triangles: onset of charge order in YBCO observed by nuclear magnetic resonance in a high magnetic field5. CDW correlations appear at or belowT** obtained from planar resistivity (Tρ**) (ref.8and Methods) and Seebeck (TS**) (Hg1201 (ref.13); YBCO19) measurements. (d) CDW correlation length (in units of the planar lattice constanta) for YBCO6,7,15,16and Hg1201. Open (solid) stars:ξ/aatTc(just belowTCDW). The maximum correlation length for YBCO is observed atp≈0.12. Dotted line: CDW modulation period 1/HCDW. Green and brown dashed lines inaandcindicateT*(p) andT**(p), respectively. (e) Temperature dependence of CDW intensity (integrated alongH) for Hg1201 obtained by RIXS (red circles) and RXD (green triangles). The CDW emerges belowTCDW=200(15) K, its intensity increases on cooling towardsTc=72 K, and then levels off (grey indicates SC phase). The CDW correlations appear well belowT*≈320 K associated withq=0 magnetic order (squares: order parameter data with representative error bars for aTc=75-K sample from ref.12), a deviation fromT-linear planar resistivity, and a considerable enhancement of AF correlations32. Inset: absence of temperature dependence ofξ/a. Vertical blue and brown bands indicateT* andT**, respectively. Figure 1a–c shows aspects of the temperature ( T ) versus doping ( p ) phase diagram of Hg1201 and YBCO, which features an insulating state with antiferromagnetic (AF) order at low hole-dopant concentrations, unusual translational-symmetry-preserving ( q =0) magnetism below the pseudogap temperature T* (refs 11 , 12 ), a Fermi-liquid regime below T** (refs 8 , 9 , 10 ) and an approximately parabolic ‘superconducting dome’ T c ( p ) (refs 13 , 14 ). The CDW correlations in YBCO are particularly prominent for hole concentrations that correspond to the ‘plateau’ in T c ( p ) (refs 6 , 7 , 15 , 16 ; Fig. 1b,c ; Supplementary Fig. 1b; Supplementary Note 1 ). Figure 1: Phase diagram. ( a ) Phase diagram of Hg1201. Blue line: T c ( p ) (ref. 13 ). Blue symbols: pseudogap (PG) temperature T *, determined from the deviation from linear- T resistivity in the ‘strange’ metallic (SM) regime and from the onset of q =0 magnetism [11] , [12] . Yellow area: Fermi-liquid (FL) regime between T ** and the measureable onset of superconducting (SC) fluctuations at T ρ ′. Grey area: estimated extent of antiferromagnetic (AF) phase. Since data below p =0.05 are unavailable for Hg1201, the phase diagram is extended to p =0 as in ref. 8 based on results for YBCO. Supplementary Fig. 1b shows comparison with YBCO. Characteristic transport temperatures are from ref. 8 and from additional measurements (see Methods). The error bar of T CDW is estimated from the CDW peak onset and marked as a brown band in e . ( b ) Solid lines: T c ( p ) for Hg1201 (ref. 13 ) and YBCO [14] . Dashed lines: hypothetical ideal (approximately parabolic) ‘superconducting domes.’ ( c ) Solid lines: deviation of the SC dome from ideal shape (multiplied by 5); p =0.09 for Hg1201 corresponds to p =0.11–0.12 for YBCO. Crosses: temperatures at which the Hall coefficient changes sign in high magnetic field [20] . Red triangles: onset of charge order in YBCO observed by nuclear magnetic resonance in a high magnetic field [5] . CDW correlations appear at or below T ** obtained from planar resistivity ( T ρ **) (ref. 8 and Methods) and Seebeck ( T S **) (Hg1201 (ref. 13 ); YBCO [19] ) measurements. ( d ) CDW correlation length (in units of the planar lattice constant a ) for YBCO [6] , [7] , [15] , [16] and Hg1201. Open (solid) stars: ξ / a at T c (just below T CDW ). The maximum correlation length for YBCO is observed at p ≈0.12. Dotted line: CDW modulation period 1 /H CDW . Green and brown dashed lines in a and c indicate T *( p ) and T **( p ), respectively. ( e ) Temperature dependence of CDW intensity (integrated along H ) for Hg1201 obtained by RIXS (red circles) and RXD (green triangles). The CDW emerges below T CDW =200(15) K, its intensity increases on cooling towards T c =72 K, and then levels off (grey indicates SC phase). The CDW correlations appear well below T* ≈320 K associated with q =0 magnetic order (squares: order parameter data with representative error bars for a T c =75-K sample from ref. 12 ), a deviation from T -linear planar resistivity, and a considerable enhancement of AF correlations [32] . Inset: absence of temperature dependence of ξ / a . Vertical blue and brown bands indicate T * and T **, respectively. Full size image We report bulk resonant X-ray-scattering measurements of Hg1201 ( p ≈0.09, T c =72 K), close to the centre of its T c ( p ) plateau. Hg1201 features a simple tetragonal crystal structure and the highest optimal superconducting transition temperature ( T c ≈97 K) of all cuprates with one CuO 2 layer per primitive cell [17] (see also Supplementary Note 2 ). For p ≈0.09, Hg1201 exhibits Fermi-liquid charge transport in zero [8] , [9] and moderate [10] magnetic fields at intermediate temperatures, as well as Shubnikov-de-Haas oscillations in high magnetic fields at temperatures well below the zero-field T c (ref. 4 ). For the present experiments, single crystals were grown and prepared according to previously described procedures [17] , [18] . Resonant X-ray scattering measurements Resonant X-ray diffraction (RXD) allows the observation of order of different electronic states of the same atomic species in a solid. For Cu L 3 -edge RXD, the spatial charge modulation of the Cu 3 d states is reflected in a modulation of the (complex) scattering factor, which gives rise to superstructure peaks at momenta corresponding to the real space periodicity. Resonant inelastic X-ray scattering (RIXS) offers the additional possibility to resolve the energy of the scattered photons, thus allowing the separation of the CDW contribution from phenomena at higher energy transfers. We quote the scattering wave vector as Q = H a *+ K b *+ L c *, where a *, b * and c * are reciprocal lattice vectors. Similar to prior work [6] , [15] , the relatively small energy of the soft X-rays constrained us to work in the first Brillouin zone. The measurements were furthermore constrained to scans of the type [ H ,0, L ], in which L was dependent on the planar momentum transfer H (see also Methods and Supplementary Fig. 2 ). 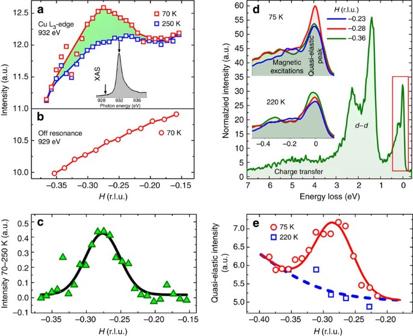Figure 2: CDW in Hg1201 (Tc=71 K) observed with RXD and RIXS. (a) RXD spectra collected near the CDW propagation vector at CuL3-resonance at 70 and 250 K. At resonance, the scattering factor becomes complex (fi′+ifi′) and strongly depends on the valence state of the resonating Cu atoms. CDW correlations give rise to the additional intensity observed at 70 K (red squares). The non-monotonic background does not change at temperatures above 200 K. The inset shows the total X-ray fluorescence spectrum (XAS) at 70 K. Arrows indicate the energies at which the momentum scans inaandbwere performed. (b) The CDW peak at 70 K is not observed off resonance. (c) Intensity difference between scans at 70 and 250 K and fit to a Gaussian function (solid line). Scans alongHandKwere found to be equivalent, as expected for the tetragonal structure of Hg1201. (d) RIXS spectra at the CuL3-edge (931.7 eV) obtained with the polarization vector perpendicular to the scattering plane (σ-polarization). Excitations typical of the cuprates are identified. The insets are zooms (red frame) for 75 and 220 K at three values ofQaround the CDW wave vector. The enhancement of the quasi-elastic peak due to the CDW is observed forHCDW≈0.28 r.l.u. The spectra are normalized to thed–dexcitation intensity. (e) Integrated intensity of the quasi-elastic peak as a function ofHat 75 and 220 K. Data are fit to a Gaussian peak with a parabolic background. The peak widths incandecorrespond to correlation length values ofξCDW/a=5.5(8) and 4.6(2), respectively. Figure 2 summarizes our observation of CDW correlations in Hg1201 via both RXD ( Fig. 2a–c ) and RIXS ( Fig. 2d,e ). RXD data were collected at the Cu L 3 -resonance (931.7 eV) with the incident beam polarized perpendicular to the scattering plane (σ-polarization). The momentum scan at 70 K ( Fig. 2a ) displays a pronounced peak that is absent away from resonance ( Fig. 2b ), which proves the involvement of the electronic degrees of freedom in the scattering process, without contribution from atomic displacements. The scan at 250 K demonstrates that CDW order is absent at this temperature ( Fig. 2b ), and only a temperature independent, non-monotonic background is observed. The peak position, H CDW =0.276(5) r.l.u., and full width at half maximum, 2 κ =0.058(9) r.l.u., at 70 K are best extracted from the intensity difference between the two temperatures ( Fig. 2c ). Figure 2: CDW in Hg1201 ( T c =71 K) observed with RXD and RIXS. ( a ) RXD spectra collected near the CDW propagation vector at Cu L 3 -resonance at 70 and 250 K. At resonance, the scattering factor becomes complex ( f i ′ + if i ′) and strongly depends on the valence state of the resonating Cu atoms. CDW correlations give rise to the additional intensity observed at 70 K (red squares). The non-monotonic background does not change at temperatures above 200 K. The inset shows the total X-ray fluorescence spectrum (XAS) at 70 K. Arrows indicate the energies at which the momentum scans in a and b were performed. ( b ) The CDW peak at 70 K is not observed off resonance. ( c ) Intensity difference between scans at 70 and 250 K and fit to a Gaussian function (solid line). Scans along H and K were found to be equivalent, as expected for the tetragonal structure of Hg1201. ( d ) RIXS spectra at the Cu L 3 -edge (931.7 eV) obtained with the polarization vector perpendicular to the scattering plane (σ-polarization). Excitations typical of the cuprates are identified. The insets are zooms (red frame) for 75 and 220 K at three values of Q around the CDW wave vector. The enhancement of the quasi-elastic peak due to the CDW is observed for H CDW ≈0.28 r.l.u. The spectra are normalized to the d – d excitation intensity. ( e ) Integrated intensity of the quasi-elastic peak as a function of H at 75 and 220 K. Data are fit to a Gaussian peak with a parabolic background. The peak widths in c and e correspond to correlation length values of ξ CDW / a =5.5(8) and 4.6(2), respectively. Full size image This finding is consistent with our RIXS experiment performed with σ-polarization and an energy resolution of 130 meV. This technique allowed the separation of the quasi-elastic peak from magnetic, 3 d inter-orbital and O 2 p /Cu 3 d charge-transfer excitations at higher energy ( Fig. 2d ). As demonstrated in ref. 6 , the quasi-elastic peak contains information about the spatial charge modulations. Figure 2d shows the low-energy inelastic spectra at three momenta for both 75 and 220 K. There is an enhancement due to CDW formation at 75 K. The full H dependence is shown in Fig. 2e . A Gaussian fit yields H CDW =0.280(5) r.l.u. and 2 κ =0.071(3) r.l.u., in very good agreement with the RXD experiment. Figure 1e shows the temperature dependence of the CDW peak intensity, obtained with the two X-ray techniques, indicating that CDW order is observed below T CDW =200(15) K. As further demonstrated in the figure, the CDW phenomenon occurs about 100 K below the onset of q =0 order [11] , [12] , which in turn coincides with T * obtained from resistivity [8] , [10] . The CDW correlations in both Hg1201 and YBCO appear at or below T **, the temperature at which the Seebeck coefficient reaches its maximum value [13] , [19] , and below which conventional Fermi-liquid planar charge transport is observed [8] , [9] , [10] (see Fig. 1a,c ; Supplementary Fig. 1b ). Recent magnetoresistance measurements revealed for tetragonal Hg1201 ( p ≈0.09 and 0.11) that Kohler’s rule is obeyed below T** , with a Fermi-liquid quasiparticle-scattering rate, in agreement with Boltzmann transport theory [10] . For YBCO, due to lower (orthorhombic) structural symmetry and the presence of Cu–O chains (along the b axis), Fermi-liquid transport is revealed only in de-twinned samples, for current flow perpendicular to the chains [8] , [10] . At least for Hg1201, the arc-like ‘Fermi surface’ (FS) should therefore be temperature independent in an extended temperature range below T **. Since the underlying Fermi-liquid regime appears to extend universally to very low hole concentrations [8] , whereas the CDW order in YBCO is most prominent for doping levels that correspond to the T c ( p ) plateau ( Fig. 1d ; Supplementary Fig. 1b ), the stable FS implied by the transport measurements for Hg1201 likely is a necessary, but not sufficient condition for the occurrence of CDW correlations. The CDW order in our Hg1201 sample is rather weak and not significantly impacted by the onset of superconductivity: the planar correlation length of ξ CDW = a /(2 πκ )≈5 a (inset in Fig. 1e ) is temperature independent and only slightly larger than the modulation period 1/ H CDW ≈3.5 a . For YBCO ( p =0.11 and 0.13 (ref. 6 )), ξ CDW takes on a similar value at high temperature, but is found to increase upon cooling towards T c : Fig. 1d shows ξ CDW both at T c and the extrapolated value at T CDW . Interestingly, ξ CDW ( p ) takes on a maximum at p =0.12, where the deviation of the T c ( p ) from a simple parabolic shape is greatest for YBCO ( Fig. 1b,c ). This deviation appears to reflect the competition between CDW order and superconductivity [2] , [6] , [7] , and the strongest suppression of the CDW amplitude in the superconducting state was observed for p =0.12 (ref. 6 ). If the magnitude of the deviation is taken as a measure of this competition, then the CDW order should be weaker in Hg1201. Indeed, we do not observe a decrease of the CDW amplitude below T c for Hg1201 close to the T c ( p ) plateau. Furthermore, we do not discern the short-range CDW order via (non-resonant) hard RXD (see Supplementary Note 3 ). In YBCO, where hard and resonant soft X-ray experiments give consistent results, the observation of CDW correlations with hard X-rays has been limited to doping levels at which the spatial correlation length is considerably larger. Given the myriad unconventional phenomena exhibited by the cuprates, especially the peculiar high-temperature ρ ~ T metallic behaviour and the opening of a pseudogap along certain portions of the FS at temperatures below T *, it came as a surprise that moderately doped YBCO exhibits QOs (ref. 3 ), the hallmark of a metal with a coherent FS. CDW correlations are considered a likely candidate for the FS reconstruction implied by the QO experiments. Nuclear magnetic resonance measurements indicate that a high magnetic field induces static long-range CDW order in YBCO [5] . The Hall, Nernst and Seebeck coefficients of YBCO and Hg1201 exhibit remarkably similar high-magnetic-field behaviour, including a low-temperature sign change, which suggests the possible existence of electron pockets as a result of the FS reconstruction [20] . The observation of QO in Hg1201 proved that pockets are indeed universally present, and not the result of the structural complexity of YBCO [4] . 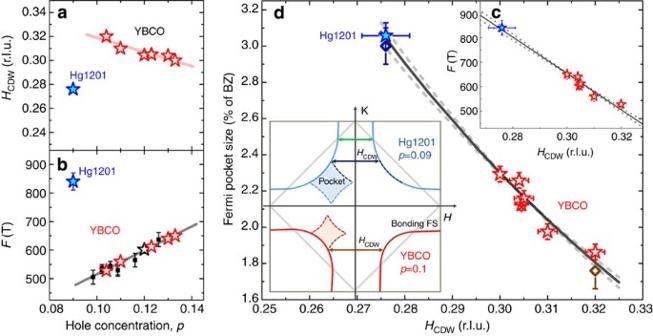Figure 3: Relationship between CDW wave vector and reconstructed Fermi pockets. (a)HCDWfor Hg1201 (blue star) and YBCO (red stars; estimated from refs6,7,15,16) as a function of hole concentration. (b) Quantum oscillation frequencyFfor Hg1201 (blue star)4and YBCO (black squares, black star)3,21as a function of hole concentration. For Hg1201, the X-ray and QO data were obtained for samples prepared under the same conditions. The black star for YBCO indicates a doping level for which both CDW and QO were measured. Red stars represent the QO frequencies estimated form the linear fit for the doping levels at which only CDW order (but not QO) was studied. (c) QO frequency versusHCDWfor Hg1201 (blue) and YBCO (red), with doping as an intrinsic parameter. The solid line represents a linear fit. The dashed lines show the fit error range. (d) Fermi-pocket size as a fraction of the first Brillouin zone versusHCDWfor Hg1201 (blue) and YBCO (red), with doping as an implicit parameter. The horizontal error bars represent the uncertainties of the CDW peak position obtained from a least-square fit of a Gaussian function to the data. The vertical error bars are estimated from the uncertainty in the QO frequency. The solid line represents a quadratic fit, which extrapolates toHCDW=0.45(2) r.l.u. in the limit of vanishing pocket size (see alsoSupplementary Note 4). The dashed lines show the fit error range. Inset: schematic of a reconstructed nodal electron pocket defined byHCDWand by the simple tight-binding Fermi surface for both Hg1201 (p=0.09 (ref.2)) and YBCO (bonding band;p=0.10, obtained from taking the average forp=0.12 (ref.7) andp=0.08 (ref.22)), with the Brillouin zone (green square) and with the AF Brillouin zone boundary (grey line). The respective pocket areas of 3.0±0.1% and 1.8±0.1% are consistent with the experiment, as indicated by dark-blue and brown diamonds ind. The green double-arrow connects the ‘hotspots’ of the tight-binding Fermi surface of Hg1201 and is substantially smaller (~0.21 r.l.u.) than the measured valueHCDW≈0.28 r.l.u. Figure 3a ( Fig. 3b ) demonstrates that the CDW modulation wave vector (QO period F ) is significantly smaller (larger) for Hg1201 than for YBCO [6] , [7] , [15] , [16] , [21] at comparable doping levels. However, if we treat the hole concentration as an implicit parameter, we find an approximately linear relationship between F and H CDW for the combined data ( Fig. 3c ) (see also Supplementary Note 4 ). On the other hand, Fig. 3d shows a fit to a plausible quadratic dependence of the fractional pocket size on H CDW , as would be expected in the simple picture of a reconstructed nodal electron pocket due to biaxial CDW order, which involves segments of the underlying FS defined by H CDW [22] . This is shown schematically in the inset to Fig. 3d , where tight-binding parameters are used to estimate the underlying FS of Hg1201 (ref. 23 ) and YBCO (bonding FS) [7] , [22] . For Hg1201, the same parametrization was recently found to be in reasonably good agreement with photoemission measurements of the nodal FS closer to optimal doping [23] . Interestingly, using the measured values of H CDW , the so-obtained pocket sizes agree with the values of the QO experiments ( Fig. 3d ). They furthermore agree with the relative values of the (negative) Hall coefficients obtained in the low-temperature, high-magnetic-field limit [20] . These observations suggest that the QO phenomenon is indeed a consequence of the universal CDW correlations. The Fermi pocket reconstructed from nodal Fermi arcs is consistent with checkerboard-type CDW order [24] , [25] and inconsistent with unidirectional charge-stripe order [26] . Our data do not allow us to test recent theoretical predictions that involve hotspots [27] , [28] or twice the anti-nodal distance [29] , since the optimal CDW wave vector does not have to connect the hotspots and because the underlying FS far from the nodal direction (in the absence of the pseudogap and CDW order) is unknown. Figure 3: Relationship between CDW wave vector and reconstructed Fermi pockets. ( a ) H CDW for Hg1201 (blue star) and YBCO (red stars; estimated from refs 6 , 7 , 15 , 16 ) as a function of hole concentration. ( b ) Quantum oscillation frequency F for Hg1201 (blue star) [4] and YBCO (black squares, black star) [3] , [21] as a function of hole concentration. For Hg1201, the X-ray and QO data were obtained for samples prepared under the same conditions. The black star for YBCO indicates a doping level for which both CDW and QO were measured. Red stars represent the QO frequencies estimated form the linear fit for the doping levels at which only CDW order (but not QO) was studied. ( c ) QO frequency versus H CDW for Hg1201 (blue) and YBCO (red), with doping as an intrinsic parameter. The solid line represents a linear fit. The dashed lines show the fit error range. ( d ) Fermi-pocket size as a fraction of the first Brillouin zone versus H CDW for Hg1201 (blue) and YBCO (red), with doping as an implicit parameter. The horizontal error bars represent the uncertainties of the CDW peak position obtained from a least-square fit of a Gaussian function to the data. The vertical error bars are estimated from the uncertainty in the QO frequency. The solid line represents a quadratic fit, which extrapolates to H CDW =0.45(2) r.l.u. in the limit of vanishing pocket size (see also Supplementary Note 4 ). The dashed lines show the fit error range. Inset: schematic of a reconstructed nodal electron pocket defined by H CDW and by the simple tight-binding Fermi surface for both Hg1201 ( p =0.09 (ref. 2 )) and YBCO (bonding band; p =0.10, obtained from taking the average for p =0.12 (ref. 7 ) and p =0.08 (ref. 22 )), with the Brillouin zone (green square) and with the AF Brillouin zone boundary (grey line). The respective pocket areas of 3.0±0.1% and 1.8±0.1% are consistent with the experiment, as indicated by dark-blue and brown diamonds in d . The green double-arrow connects the ‘hotspots’ of the tight-binding Fermi surface of Hg1201 and is substantially smaller (~0.21 r.l.u.) than the measured value H CDW ≈0.28 r.l.u. Full size image Recent combined RXD and scanning-tunneling microscopy work demonstrated the presence of CDW correlations in both Bi 2 Sr 2− x La x CuO 6+ δ (Bi2201) (ref. 27 ) and Bi 2 Sr 2 CaCu 2 O 8+ δ (Bi2212) (ref. 30 ), with values of H CDW between 0.25 and 0.30 r.l.u., consistent between the bulk (RXD) and surface (scanning-tunneling microscopy) techniques. Similar to the present result for Hg1201, ξ CDW was found to be rather small (~7 a ). Whereas YBCO exhibits a clear anti-correlation between CDW and superconducting order, for single-layer Bi2201 and double-layer Bi2212 the RXD signal is not significantly suppressed below T c . All three cuprates exhibit lower structural symmetry than Hg1201, and therefore are less ideal for a quantitative study of the connection between charge transport and CDW order [31] . Although QOs below optimal doping were first discovered in YBCO [3] , pristine planar Fermi-liquid transport ( ρ ~ T 2 in zero magnetic field; confirmed by the validity of Kohler’s rule for the magnetoresistance) is only found for current flow perpendicular to the Cu–O chains [8] , [10] . Bi2201 and Bi2212 are more disordered [31] , which has prevented the observation of pristine Fermi-liquid transport, including QO. For Bi2201, a direct correlation between H CDW and the distance between the Fermi-arc tips was suggested based on combined photoemission and X-ray work [27] . Whereas ref. 30 suggests that pseudogap formation precedes CDW order in Bi2212, consistent with our finding, it is argued in ref. 27 that T CDW ≈ T * for Bi2201. However, given the statistical uncertainty in the RXD data for Bi2201, the appearance of CDW order may also be interpreted to coincide with T **. The present work provides strong support for the idea that incommensurate CDW correlations drive the FS reconstruction implied by the QO experiments. Moreover, it demonstrates that much can be learned from a comparative study of Hg1201 with other cuprates, and especially with YBCO. Whereas interpretation of results for YBCO is complicated by the orthorhombic double-CuO 2 -layer structure [8] , [10] , [22] , the situation for Hg1201 is more straightforward. Neutron-scattering experiments have demonstrated universal q =0 magnetism [11] along with a significant build-up of gapped AF correlations [32] upon the formation of the pseudogap at T *. The combined results are consistent with the possibility that the sequence of ordering tendencies ( q =0 order precedes CDW order, which in turn precedes superconducting order) and the phase diagram as a whole are driven by short-range AF correlations [26] , [28] , [33] , [34] . Sample preparation Hg1201 single crystals were grown by a two-step flux method [18] , subsequently annealed at 400 °C in partial vacuum of 100 mtorr [17] and then quenched to room temperature. The width of the superconducting transition, as determined from magnetic susceptibility, was typically 2 K with a midpoint of T c =72 K. According to the T c versus p relationship established for polycrystalline samples [13] , this corresponds to a hole concentration of p ≈0.09. The typical sample mosaicity, measured with hard RXD via rocking curve at several ( H 0 0)-type Bragg reflection, was 0.030(2) deg. The typical crystal dimensions were 2 × 2 × 0.5 mm 3 . The X-ray penetration length in Hg1201 is about 0.2 μm at the energy used in the soft X-ray experiment ( ℏ ω ≈932 eV). To ensure a flat and clean surface, each sample was polished multiple times with sandpaper with increasingly finer grade, ranging from 1 to 0.05 μm. The same sample preparation process was used in separate X-ray absorption spectroscopy characterizations of Hg1201 at O K and Cu L 3 edges, giving us high confidence that the procedure does not change the hole concentration. Resistivity characterization (four-point measurements in the temperature range 4–350 K) for a sample from the same batch and for an additional T c =90-K sample ( p ≈0.12) was performed with a Quantum Design, Inc., Physical Properties Measurement System. The samples were prepared and measured, and the corresponding characteristic temperatures (included in Fig. 1a ; Supplementary Fig. 1b ) and error bars were obtained according to the procedure described in ref. 8 . Experimental set-up Resonant X-ray-scattering techniques combine the sensitivity of traditional RXD to ordered structures with the advantages of site-selective X-ray absorption spectroscopy. By tuning the incident photon energy to match the Cu L 3 -edge, the CuO 2 layers can be studied directly through excitations of core 2 p 3/2 electrons into the Cu 3 d valence band, with a high sensitivity to spatial charge modulations. RXD measurements at the Cu L 3 -edge were performed at the UE46-PGM1 beam line of the BESSY-II synchrotron in Berlin, Germany [35] . To determine the exact resonance energy, X-ray absorption measurements were performed in a total fluorescence yield configuration. The incident X-ray beam was then tuned to the maximum of the fluorescence signal at ℏ ω =931.7 eV. Since the structure of Hg1201 contains only one Cu site, a fluorescence spectrum displays a single maximum (inset to Fig. 2a ). The momentum scans were performed by rotating the sample about the axis perpendicular to the scattering plane, and the detector angle was set to 2 θ =160 deg. The maximum in-plane momentum-transfer component (the projection of the momentum vector onto the CuO 2 plane; see Supplementary Fig. 2 ) at 931.7 eV was q =±0.42 r.l.u. In the configuration used in the experiment, K was set to zero, and H was coupled to L during the scans. The maximum of the CDW peak was observed at H =−0.28 r.l.u., with L =1.25 r.l.u. RIXS measurements were carried out at the ADRESS beam line [36] of the Swiss Light Source, Paul Scherrer Institut, Villigen, Switzerland. The SAXES spectrometer [37] with a fixed scattering angle 2 θ =130 deg was employed. Similar to the RXD experiment, momentum scans were performed by rotating the sample about the axis perpendicular to the scattering plane. The maximum accessible in-plane component of the momentum transfer was q =±0.38 r.l.u. With K set to zero, the maximum of the CDW peak was observed at H =−0.28 r.l.u. In our scattering geometry, the maximum corresponded to L =1.12 r.l.u. The energy spectrum of the scattered intensity was analysed by a grating and recorded with a two-dimensional charge-coupled device detector. The energy resolution was 130 meV, as determined from a measurement of the elastic peak of polycrystalline graphite away from the carbon resonance. At each momentum transfer, the energy-loss spectrum was measured five times, each with a 10-min collecting time. The momentum dependence of the quasi-elastic peak (at zero energy loss) was analysed as a function of momentum transfer. Each energy loss scan was normalized to the total inelastic intensity above the energy loss of 0.8 eV. Most of the RIXS measurements were carried out with incident polarization perpendicular to the scattering plane (σ-polarization), and with a negative in-plane component of the momentum transfer vector ( Supplementary Fig. 2 ), as this resulted in a larger signal. As demonstrated in ref. 6 , the cross-section for charge and spin excitations is polarization dependent. For positive in-plane momenta, the intensity of spin excitations increases relative to that of the charge excitations upon switching the polarization from σ to π (polarization vector parallel to the scattering plane). We observed no increase of the intensity as the polarization was changed from σ to π, and therefore can rule out that the observed signal is magnetic. Temperature dependence The temperature dependence of the CDW peak was studied primarily with the RXD technique. Momentum scans were performed in the temperature range from 4 to 280 K. The data were collected on increasing the temperature with a constant ramp of 1 K min −1 , and every scan corresponded to a temperature change of 1 K. Every four consecutive scans were averaged during the data analysis for further processing. To obtain the temperature-dependent contribution to the scattered intensity, the background scattering at 250 K was subtracted from every scan. The background-subtracted data were fit with a Gaussian function. Data collected at a number of temperatures, as well as the temperature dependence of the peak amplitude and width are presented in Supplementary Fig. 4 . The error bars in Fig. 1e represent the uncertainty of the Gaussian fit to the CDW peak area. In the inset, the error bars are the uncertainties of the fitted widths. RIXS measurements were performed at five temperatures between 10 and 220 K. The temperature dependences of the CDW peak obtained by the two techniques are in excellent agreement. How to cite this article: Tabis, W. et al. Charge order and its connection with Fermi-liquid charge transport in a pristine high- T c cuprate. Nat. Commun. 5:5875 doi: 10.1038/ncomms6875 (2014).